Transcriptional repression by the HDAC4–RelB–p52 complex regulates multiple myeloma survival and growth Although transcriptional activation by NF-κB is well appreciated, physiological importance of transcriptional repression by NF-κB in cancer has remained elusive. Here we show that an HDAC4–RelB–p52 complex maintains repressive chromatin around proapoptotic genes Bim and BMF and regulates multiple myeloma (MM) survival and growth. Disruption of RelB–HDAC4 complex by a HDAC4-mimetic polypeptide blocks MM growth. RelB-p52 also represses BMF translation by regulating miR-221 expression. While the NIK-dependent activation of RelB-p52 in MM has been reported, we show that regardless of the activation status of NIK and the oncogenic events that cause plasma cell malignancy, several genetically diverse MM cells including Bortezomib-resistant MM cells are addicted to RelB-p52 for survival. Importantly, RelB is constitutively phosphorylated in MM and ERK1 is a RelB kinase. Phospho-RelB remains largely nuclear and is essential for Bim repression. Thus, ERK1-dependent regulation of nuclear RelB is critical for MM survival and explains the NIK-independent role of RelB in MM. Multiple Myeloma (MM) is a monoclonal tumour of plasma cells (PCs) that develops from post germinal-center (GC) B cells [1] , [2] . While MM tumours have been classified into different genetic subgroups based on several genetic abnormalities [1] , [2] , [3] , [4] , [5] , [6] , [7] , several of them are divided into three distinct groups of chromosomal translocations involving (1) Cyclin D (2) MAF and (3) MMSET/FGFR3 genes [2] . To develop novel therapeutic approaches to target all the genetic subgroups of MM, it is important to identify the molecular requirements and the survival signals that are common to all genetic subgroups of MM tumours. Among the genetic abnormalities found in MM, activating mutations of the RAS and BRAF pathway, dysregulation of the myc gene and activating mutations in the NF-κB pathway have been frequently observed [2] , [6] . Of these, the NF-κB pathway is of particular significance in the pathogenesis of MM because NF-κB not only provides survival and proliferation signals to the MM tumours but also promotes the release of several cytokines that further enhance tumour growth. Mammalian NF-κB is activated by two distinct pathways namely the IKKβ-dependent classical (RelA-p50) pathway and the NF-κB inducing kinase (NIK) and IKKα-dependent alternative (RelB-p52) pathway [8] , [9] . Although, NF-κB is frequently activated in cancer [9] , the mechanism by which NF-κB contributes to tumour growth is likely to be different in different tumours [9] , [10] , [11] , [12] , [13] , [14] . Importantly, while transcriptional activation by NF-κB is well appreciated [8] , [15] , [16] , [17] , [18] , [19] , the physiological significance of transcriptional repression by NF-κB in cancer has not been established. While maintenance of pro-tumorigenic repressive chromatin in cancer has been well described [19] , [20] , [21] , it is not clear whether NF-κB is essential for maintaining repressive chromatin that facilitates tumour growth. Moreover, while transcriptionally active complexes formed by NF-κB are extensively studied [22] , the molecular nature of transcriptionally repressive NF-κB complexes is not well established. Identification of novel gene regulatory NF-κB complexes that are essential for the maintenance of repressive chromatin and tumour growth will enable us to develop novel therapeutic approaches for cancer cure. Classical NF-κB complexes (RelA-p50) have been well studied for their role in tumour survival and growth, but the relative contribution of the alternative NF-κB (RelB-p52) in cancer has been unclear. In MM, both classical and the alternative pathways were reported to be active due to various mutations [23] , [24] . Among these, mutations in the genes encoding TRAF3, TRAF2 and combined loss of cIAP1 and cIAP2 leading to the stabilization and activation of NIK, were frequently found in MM [24] . Stabilization of NIK leads to constitutive processing of p100 to p52 and activation of the alternative RelB-p52 pathway [25] , [26] . While NIK was found to be dispensable for the activation of IKKβ-dependent classical pathway [27] , [28] , in MM, NIK stabilization was shown to activate the classical pathway presumably due to direct interaction between NIK and IKKβ [23] . Surprisingly, RNAi-mediated silencing of IKKα, the kinase through which NIK activates the alternative NF-κB pathway [8] , [29] did not influence the survival of MM cells [23] , whereas pharmacological inhibition of IKKβ in MM cells harbouring NIK stabilizing mutations led to apoptosis [23] . Another report suggested that targeting IKKα impairs MM tumour growth without influencing NF-κB activation [30] . Collectively, these reports suggested that downstream of NIK, activation of IKKβ-dependent classical NF-κB plays an important role in MM-cell survival whereas the role of IKKα-dependent RelB-p52 pathway in MM remained elusive. The proteasome machinery, which plays a critical role in NF-κB signalling has been a major target for MM treatment [31] , [32] and Bortezomib, a proteasome inhibitor, has been used as a potent anti-MM drug in the clinic [33] . However, development of resistance to Bortezomib has been a major problem in MM therapy [34] , [35] . Thus, it is necessary to identify novel molecular targets that are necessary for the survival of both parental and Bortezomib resistant MM cells. Interestingly, recent reports indicate that combined use of histone deacetylase (HDAC) inhibitors and proteasome inhibitors seems to be a promising approach for the treatment of relapsed MM [36] . While some reports indicated HDAC3 and HDAC6 as attractive drug targets in MM [37] , [38] , it is not clear which HDAC is commonly required for the survival of most genetic subgroups of MM cells. Here we report that a novel HDAC4–RelB–p52 complex maintains repressive chromatin around proapoptotic genes BMF and Bim and is essential for the survival and growth of several genetically diverse MM cell lines (MMCLs) as well as for colony formation by MM progenitor cells. Importantly, disruption of the RelB–HDAC4 complex by a short HDAC4-mimetic polypeptide was sufficient to induce Bim and impair MM tumour growth in vivo . Our data further indicate that several genetically diverse MM cells, including Bortezomib-resistant MM cells are addicted to RelB–p52 for survival, regardless of the activation status of NIK/IKK and the oncogenic events that caused the malignancy. While the cytoplasmic regulation of RelB has been well studied [8] , nuclear regulation of RelB by posttranslational modifications affecting its transcriptional function has remained elusive. Here we show that RelB is constitutively phosphorylated in most MMCLs as well as in human patient derived primary MM cells and that phospho-RelB is primarily localized to the nucleus. Importantly, we found that ERK1 is a novel RelB-kinase and that ERK1-mediated RelB phosphorylation is essential for Bim repression and MM cell survival. Collectively, our data indicate that a novel nuclear regulatory mechanism involving ERK1-mediated RelB phosphorylation and transcriptional repression by HDAC4–RelB–p52 plays an essential role in MM cell survival. Further, our results suggest that HDAC4–RelB–p52 is an important molecular target for developing novel therapeutic approaches for MM treatment. RelB-p52 addiction in multiple myeloma In a subset of MMCLs, mutations leading to NIK stabilization (here after mentioned as NIK high ) were reported [23] . Surprisingly, within these NIK high MMCLs, IKKβ, a kinase that regulates the classical RelA-p50 pathway was shown to be essential for survival, whereas depletion of IKKα, an essential kinase for RelB-p52 activation had no effect on MM cell survival [23] . However, many of these NIK high MMCLs displayed high levels of nuclear RelB-p52 complexes ( Supplementary Fig. 1 ) [23] whose role in MM remained unclear. This prompted us to directly investigate the function of RelB-p52 in MM. To this end, we employed sh-RNA mediated silencing of RelB or NF-kB2 and found that both RelB and NF-κB2 (p52) are essential for the survival of several MMCLs ( Fig. 1a , Supplementary Fig. 1a ). Interestingly, RelB and p52 were essential for the survival of several genetically diverse MM cells, regardless of the activation status of NIK or IKK and regardless of the oncogenic events that caused the malignant transformation of plasma cells ( Fig. 1a ). Moreover, in our analysis we included three distinct groups of MMCLs with regards to NF-κB activation: (1) ‘Alternative NF-κB’: MMCLs with mutations leading to stabilization and activation of NIK; (2) ‘Classical NF-κB’: activation of IKKβ; (3) ‘None’: MMCLs that does not harbour mutations known to stabilize NIK or activate IKKβ ( Supplementary Fig. 1b ). In all three groups of MMCLs, however, some basal levels of RelB-p52 were seen in the nucleus and depletion of RelB-p52 subjected all three groups of MMCLs to apoptosis ( Fig. 1a , Supplementary Fig. 1b ). This indicated that even in the absence of active NIK, some basal activity of RelB-p52 is essential for the survival of several genetically diverse MMCLs ( Fig. 1a , Supplementary Fig. 1b ). Two different sh-RNAs targeting RelB or NF-kB2 were employed and generated similar results ( Supplementary Fig. 1a ). In line with their requirement for survival of MM cells in vitro , depletion of RelB or NF-κB2 completely impaired the growth of human MM xenografts in vivo in nude mice ( Fig. 1b,c ). Importantly, as shown in Fig. 1d,e and Supplementary Fig. 1c,d , depletion of RelB or NF-κB2 severely impaired colony formation by MM progenitor cells in semisolid methyl-cellulose cultures. This result is of particular significance, because it was previously shown that the MM tumour progenitor cells are relatively resistant to Bortezomib treatment [39] , [40] . This result prompted us to test whether RelB-p52 are essential for the survival of Bortezomib-resistant MM cells. To this end, we depleted RelB in Bortezomib-resistant RPMI-8226 cells and found that RelB is essential for the survival of not only parental, but also Bortezomib-resistant MM cells ( Fig. 1a,f ). To ensure that apoptosis of MM cells upon RelB-depletion was not due to off-target effects of sh-RNA, we infected KMM1 cells with a lentiviral vector that simultaneously expresses (1) sh-RNA targeting the 3′-UTR of endogenous RelB mRNA and (2) exogenous RelB cDNA that is resistant to RelB specific sh-RNA ( Supplementary Fig. 1e ). As shown in Fig. 1g and Supplementary Fig. 1f–h , presence of exogenous sh-resistant RelB completely rescued KMM1 cells from apoptosis induced by depletion of endogenous RelB. Interestingly, RelB-depletion did not affect survival of non-Hodgkin’s lymphoma (NHL) cells ( Supplementary Fig. 1i ) suggesting a unique requirement of RelB-p52 for the survival of several genetically diverse MMCLs as well as Bortezomib resistant MM cells, indicating an addiction towards RelB-p52 in MM. 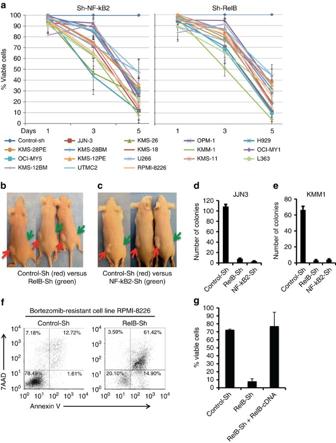Figure 1: RelB-p52 addiction in multiple myeloma (MM). (a) Indicated MM cell lines were infected with lentiviruses expressing control-Sh RNA or sh-RNAs targeting RelB or NF-kB2 and apoptosis was measured by flow-cytometry on staining with 7AAD and Annexin-V and % viable cells were plotted as indicated. For convenience, % viable cells for control-Sh was measured as 100% and the viability in RelB- and NF-κB2-depleted cells was normalized accordingly. (b,c) JJN3 cells were infected with lentiviruses expressing control-sh RNA or sh-RNAs targeting RelB or NF-kB2. On day 2 post infection, cell viability was measured to be equal among control, RelB and NF-κB2-depleted cells and 3 × 106cells were subcutaneously injected into nude mice. Tumour growth was analysed as indicated. Red arrows indicate injection of control-Sh expressing cells on the left side and Green arrows indicate RelB or NF-κB2-depleted cells on the right side. Note the complete block in MM tumour growth on RelB or NF-κB2 depletion. A representative figure from three experimental replicates (n=3 in each experiment) is shown. (d,e) JJN3 and KMM1 cells were infected with lentiviruses expressing the indicated sh-RNAs and 24 h later equal number of cells (2000) were seeded into semisolid methyl-cellulose cultures. Colony formation was followed for about 10 days and the number of colonies was presented as indicated. (f) Bortezomib resistant RPMI-8226 cells were infected with lentiviruses expressing the indicated sh-RNAs and apoptosis was measured by flow-cytometry as explained above. (g) KMM1 cells were infected with lentiviruses expressing control-Sh RNA, RelB-Sh RNA targeting the 3′-UTR of RelB or a lentivirus simultaneously expressing a 3′-UTR specific RelB-Sh RNA and RelB cDNA that is resistant to RelB-Sh RNA. Five days after infection apoptosis was measured by flow-cytometry as explained above and the % viable cells were plotted as indicated. Error bars indicate s.d.n=3. Representative figures from —Three to five experimental replicates are shown. Figure 1: RelB-p52 addiction in multiple myeloma (MM). ( a ) Indicated MM cell lines were infected with lentiviruses expressing control-Sh RNA or sh-RNAs targeting RelB or NF-kB2 and apoptosis was measured by flow-cytometry on staining with 7AAD and Annexin-V and % viable cells were plotted as indicated. For convenience, % viable cells for control-Sh was measured as 100% and the viability in RelB- and NF-κB2-depleted cells was normalized accordingly. ( b , c ) JJN3 cells were infected with lentiviruses expressing control-sh RNA or sh-RNAs targeting RelB or NF-kB2. On day 2 post infection, cell viability was measured to be equal among control, RelB and NF-κB2-depleted cells and 3 × 10 6 cells were subcutaneously injected into nude mice. Tumour growth was analysed as indicated. Red arrows indicate injection of control-Sh expressing cells on the left side and Green arrows indicate RelB or NF-κB2-depleted cells on the right side. Note the complete block in MM tumour growth on RelB or NF-κB2 depletion. A representative figure from three experimental replicates ( n =3 in each experiment) is shown. ( d , e ) JJN3 and KMM1 cells were infected with lentiviruses expressing the indicated sh-RNAs and 24 h later equal number of cells (2000) were seeded into semisolid methyl-cellulose cultures. Colony formation was followed for about 10 days and the number of colonies was presented as indicated. ( f ) Bortezomib resistant RPMI-8226 cells were infected with lentiviruses expressing the indicated sh-RNAs and apoptosis was measured by flow-cytometry as explained above. ( g ) KMM1 cells were infected with lentiviruses expressing control-Sh RNA, RelB-Sh RNA targeting the 3′-UTR of RelB or a lentivirus simultaneously expressing a 3′-UTR specific RelB-Sh RNA and RelB cDNA that is resistant to RelB-Sh RNA. Five days after infection apoptosis was measured by flow-cytometry as explained above and the % viable cells were plotted as indicated. Error bars indicate s.d. n =3. Representative figures from —Three to five experimental replicates are shown. Full size image Transcriptional repression of BMF and Bim genes by RelB-p52 To investigate the mechanism by which RelB-p52 regulate survival of MM cells, we analysed the expression levels of several Bcl-2 family members. While we did not find significant changes in the levels of several anti- and proapoptotic members of the Bcl2 family ( Supplementary Fig. 2a,b ), we repeatedly observed highly elevated levels of BMF and Bim upon depletion of RelB or NF-κB2 in different MMCLs ( Fig. 2a–c , Supplementary Fig. 2c–e ). Two different sh-RNAs were employed and obtained similar results ( Fig. 2c , Supplementary Fig. 2c ). RelB-depletion also resulted in elevated levels of Bim in Bortezomib resistant MM cells ( Fig. 2d ) suggesting that RelB-regulation of Bim repression is an important survival mechanism operated in MM. We next investigated whether RelB-p52 directly regulate BMF and Bim gene promoters. To this end, by employing bio-informatic methods, we first analysed 2.5-kb regions upstream of human BMF and Bim genes and found the presence of few potential NF-κB binding sites ( Supplementary Fig. 2f,g ). We then cloned the 2.5 kb promoters of BMF and Bim genes into pGL2 basic luciferase reporter vector and analysed their regulation by RelB-p52. As shown in Supplementary Fig. 2h,i , co-transfection of RelB and p52 in HEK-293T cells resulted in significant repression of promoter activity of both Bim and BMF genes. To confirm that RelB-p52 regulate Bim and BMF genes by directly being recruited to their promoters, we employed chromatin immunoprecipitation (ChIP) assay and found that both RelB and p52 are recruited to a potential NF-κB binding site (−146 to −300) in Bim and (−4 to −164) in BMF - gene promoters in MM cells ( Fig. 2e,f ). RelB and p52 were also recruited to other proximal NF-κB sites but not to a non-specific region located about 2 kb further upstream (−2476 to −2201) within the Bim promoter ( Fig. 2e lower panel) indicating selective recruitment of RelB-p52 to distinct binding sites. Importantly, RelB was recruited to the Bim promoter not only in MMCLs in which NIK was stabilized (NIK high ) but also in MMCLs such as KMS-28BM, H929 and OPM1, in which NIK levels were invisible (here after mentioned as NIK low ; Fig. 2e , Supplementary Fig. 2j and Supplementary Fig. 1b ) suggesting that the basal level of nuclear RelB in NIK low cell lines is sufficient to bind and repress Bim promoter and that depletion of RelB-p52 in NIK low cell lines also results in elevated levels of Bim and apoptosis ( Supplementary Fig. 2e,d , Fig. 1a ). 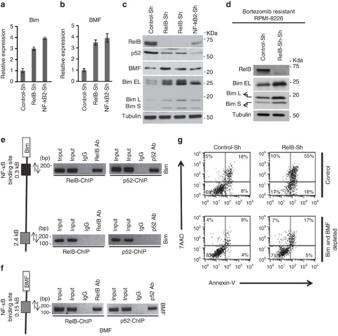Figure 2: Transcriptional repression ofBimandBMFgenes by RelB-p52. (a,b) Total RNA from JJN3 cells infected with lentiviruses expressing Control-Sh RNA or sh-RNAs targeting RelB or NF-kB2 was analysed by qRT–PCR for the expression of Bim and BMF. (c,d) Whole cell lysates from JJN3 cells and Bortezomib resistant RPMI-8226 cells infected with lentiviruses expressing the indicated sh-RNAs, were analysed for the indicated proteins by immunoblotting. (e,f) Recruitment of RelB and p52 to the endogenous Bim and BMF promoters. Chromatin from JJN3 cells was immunoprecipitated using α-RelB or α-p52 antibodies. Normal IgG was used as a control. Recruitment of RelB and p52 to theBim(e) andBMF(f) promoters was analysed by PCR-amplification of the immunoprecipitated DNA using specific primers that amplified a 154-bp region (−300 to −146) close to theBimgene transcriptional start site and a 160-bp region (−164 to −4) proximal to theBMFtranscriptional start site. As a control, a region spanning −2476 to −2201 of theBimpromoter was also amplified using primers specific to this region (elower panel). Amplified PCR products were analysed by running on agarose gels as indicated. Note that RelB-p52 were recruited specifically to a site that is 300 bp upstream but not to a region that is 2.4-kb upstream to theBimtranscriptional start site. (g) Combined depletion of Bim and BMF rescues RelB-depleted cells from apoptosis. JJN3 cells were infected with lentiviruses expressing control Sh-RNA or Sh-RNAs targeting Bim and BMF and were selected in puromycin prior to silencing RelB. Apoptosis was measured as explained above. Note the significant rescue from apoptosis of RelB-silenced cells in the absence of Bim and BMF. Error bars indicate s.d.n=3. Representative figures from —three to five experimental replicates are shown. Figure 2: Transcriptional repression of Bim and BMF genes by RelB-p52. ( a , b ) Total RNA from JJN3 cells infected with lentiviruses expressing Control-Sh RNA or sh-RNAs targeting RelB or NF-kB2 was analysed by qRT–PCR for the expression of Bim and BMF. ( c , d ) Whole cell lysates from JJN3 cells and Bortezomib resistant RPMI-8226 cells infected with lentiviruses expressing the indicated sh-RNAs, were analysed for the indicated proteins by immunoblotting. ( e , f ) Recruitment of RelB and p52 to the endogenous Bim and BMF promoters. Chromatin from JJN3 cells was immunoprecipitated using α-RelB or α-p52 antibodies. Normal IgG was used as a control. Recruitment of RelB and p52 to the Bim ( e ) and BMF ( f ) promoters was analysed by PCR-amplification of the immunoprecipitated DNA using specific primers that amplified a 154-bp region (−300 to −146) close to the Bim gene transcriptional start site and a 160-bp region (−164 to −4) proximal to the BMF transcriptional start site. As a control, a region spanning −2476 to −2201 of the Bim promoter was also amplified using primers specific to this region ( e lower panel). Amplified PCR products were analysed by running on agarose gels as indicated. Note that RelB-p52 were recruited specifically to a site that is 300 bp upstream but not to a region that is 2.4-kb upstream to the Bim transcriptional start site. ( g ) Combined depletion of Bim and BMF rescues RelB-depleted cells from apoptosis. JJN3 cells were infected with lentiviruses expressing control Sh-RNA or Sh-RNAs targeting Bim and BMF and were selected in puromycin prior to silencing RelB. Apoptosis was measured as explained above. Note the significant rescue from apoptosis of RelB-silenced cells in the absence of Bim and BMF. Error bars indicate s.d. n =3. Representative figures from —three to five experimental replicates are shown. Full size image To confirm that the apoptosis upon RelB-p52 depletion was due to elevation in the levels of Bim and BMF, we first depleted both Bim and BMF and examined the effect of RelB silencing in Bim- and BMF-depleted cells ( Fig. 2g , Supplementary Fig. 2k ). As shown in Fig. 2g , combined loss of Bim and BMF resulted in a significant rescue of RelB-depleted cells from apoptosis. Further, expression of moderate levels of exogenous BMF caused apoptosis in JJN3 cells ( Supplementary Fig. 2l,m ). Collectively, these results indicate that transcriptional repression of Bim and BMF genes by RelB-p52 is a novel survival strategy operated in MM. Interaction of RelB with HDAC4 in MM How RelB-p52 repress gene transcription is not clear. To this end, we searched for RelB interacting transcriptional repressors in MM cells and found that endogenous RelB frequently interacts with HDAC4 in different MMCLs including JJN3, KMM1 and JK6L cells ( Fig. 3a , Supplementary Fig. 3 ). Moreover, upon cotransfection in HEK-293T cells, we found that RelB and HDAC4 interact with each other ( Fig. 3b,c ). Further, immunoprecipitation of endogenous p52 resulted in co-immunoprecipitation of both RelB and HDAC4 indicating that HDAC4, RelB and p52 exist in one complex ( Fig. 3d ). Collectively, these results indicate the formation of a novel HDAC4–RelB–p52 complex in MM cells. 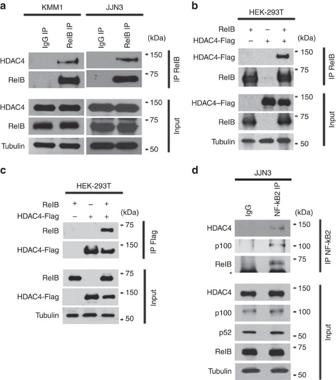Figure 3: RelB-p52 interaction with HDAC4 in MM. (a) Endogenous RelB was immunoprecipitated from whole cell lysates of KMM1 and JJN3 cells and its interaction with HDAC4 was analysed by immunoblotting as indicated. (b) HEK-293T cells were cotransfected with RelB and HDAC4-Flag and their interaction was analysed by immunoblotting on immunoprecipitation of RelB (b) or HDAC4-Flag (c) using α-RelB or α-Flag antibodies as indicated. Immunoprecipitates were probed for the indicated proteins by immunoblotting. (d) Endogenous p52 was immunoprecipitated from JJN3 cells using anti-NF-κB2 antibody and the immunoprecipitates were analysed for HDAC4, RelB and p100 by immunoblotting. Input lysates in (a–d) were probed for the indicated proteins by immunoblotting. *immunoglobulin band. Representative figures from 3 experimental replicates are shown. Figure 3: RelB-p52 interaction with HDAC4 in MM. ( a ) Endogenous RelB was immunoprecipitated from whole cell lysates of KMM1 and JJN3 cells and its interaction with HDAC4 was analysed by immunoblotting as indicated. ( b ) HEK-293T cells were cotransfected with RelB and HDAC4-Flag and their interaction was analysed by immunoblotting on immunoprecipitation of RelB ( b ) or HDAC4-Flag ( c ) using α-RelB or α-Flag antibodies as indicated. Immunoprecipitates were probed for the indicated proteins by immunoblotting. ( d ) Endogenous p52 was immunoprecipitated from JJN3 cells using anti-NF-κB2 antibody and the immunoprecipitates were analysed for HDAC4, RelB and p100 by immunoblotting. Input lysates in ( a – d ) were probed for the indicated proteins by immunoblotting. *immunoglobulin band. Representative figures from 3 experimental replicates are shown. Full size image HDAC4–RelB–p52 complex maintains repressive chromatin Although the above results demonstrated formation of an HDAC4–RelB–p52 complex, its physiological relevance to the repression of BMF and Bim genes was not clear. We therefore, investigated whether HDAC4 is recruited to the BMF and Bim gene promoters by ChIP analysis and found that similar to RelB and p52, HDAC4 is also recruited to the regions corresponding to −164 to −4 on BMF and −300 to −146 on Bim gene promoters ( Fig. 4a,b left panels, Supplementary Fig. 4a ). Importantly, depletion of RelB completely impaired HDAC4 recruitment to both Bim and BMF gene promoters indicating that RelB recruits HDAC4 to the promoters of these genes ( Fig. 4a,b middle panels). Moreover, depletion of RelB resulted in increased histone acetylation around Bim and BMF gene promoters as indicated by the ChIP analysis of acetyl-Histone H3 occupancy on these promoters ( Fig. 4a,b right panels). Collectively these results indicate that HDAC4–RelB–p52 complex maintains repressive chromatin on Bim and BMF gene promoters by keeping the histones in a deacetylated state. 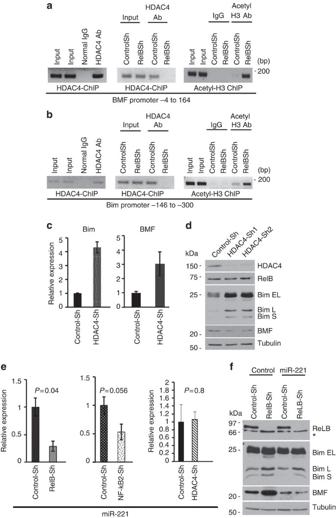Figure 4: RelB recruits HDAC4 and maintains repressive chromatin onBimandBMFpromters. Chromatin from control or RelB-depleted JJN3 cells was immunoprecipitrated with α-HDAC4, α-Acetyl H3 or normal IgG antibodies. Recruitment of HDAC4 to theBMF(a) andBim(b) promoters (aandbleft and middle panels) was analysed by PCR-amplification of the immunoprecipitated DNA using specific primers corresponding toBMFandBimpromoters. Note the loss of HDAC4 recruitment in the absence of RelB. Acetylation of Histone H3 onBMFandBimpromoters was analysed by ChIP assay using α-acetyl H3 antibody and PCR-amplification of immunoprecipitated DNA as explained above (aandbright panels). (c) Increased expression of proapoptotic Bim and BMF genes on HDAC4 depletion. Total RNA from JJN3 cells infected with lentiviruses expressing Control-Sh RNA or sh-RNA targeting HDAC4, was analysed by quantitative PCR for the expression of Bim and BMF and relative expression was plotted as indicated. (d) Increase in proapoptotic Bim but not BMF protein levels on HDAC4 depletion. Whole cell lysates from JJN3 cells infected with lentiviruses expressing indicated sh-RNAs, were analysed for the indicated proteins by immunoblotting. Note the elevation of Bim but not BMF protein levels on depletion of HDAC4. (e) RelB-p52 regulation of miR-221 in MM cells. RNA from JJN3 cells infected with lentiviruses expressing Control-sh RNA or sh-RNAs targeting RelB, NF-kB2 or HDAC4 were analysed by quantitative PCR for miR-221 expression. Note the down regulation of miR-221 on RelB or NF-κB2 depletion but not on HDAC4-depletion. (f) Exogenous miR-221 prevents elevation of BMF protein levels in RelB-depleted cells. JJN3 cells infected with control or miR-221 expressing lentiviruses were superinfected with lentiviruses expressing control-Sh RNA or sh-RNA targeting RelB. Whole cell lysates were analysed by immunoblotting for the indicated proteins. Note the elevation of Bim protein levels in RelB depleted cells in both control and miR-221 overexpressing cells, whereas BMF protein levels were increased only in RelB depleted control but not in miR-221 over expressing cells. *non-specific band. Error bars indicate s.d.n=3. Representative figures from 3 experimental replicates are shown. Figure 4: RelB recruits HDAC4 and maintains repressive chromatin on Bim and BMF promters. Chromatin from control or RelB-depleted JJN3 cells was immunoprecipitrated with α-HDAC4, α-Acetyl H3 or normal IgG antibodies. Recruitment of HDAC4 to the BMF ( a ) and Bim ( b ) promoters ( a and b left and middle panels) was analysed by PCR-amplification of the immunoprecipitated DNA using specific primers corresponding to BMF and Bim promoters. Note the loss of HDAC4 recruitment in the absence of RelB. Acetylation of Histone H3 on BMF and Bim promoters was analysed by ChIP assay using α-acetyl H3 antibody and PCR-amplification of immunoprecipitated DNA as explained above ( a and b right panels). ( c ) Increased expression of proapoptotic Bim and BMF genes on HDAC4 depletion. Total RNA from JJN3 cells infected with lentiviruses expressing Control-Sh RNA or sh-RNA targeting HDAC4, was analysed by quantitative PCR for the expression of Bim and BMF and relative expression was plotted as indicated. ( d ) Increase in proapoptotic Bim but not BMF protein levels on HDAC4 depletion. Whole cell lysates from JJN3 cells infected with lentiviruses expressing indicated sh-RNAs, were analysed for the indicated proteins by immunoblotting. Note the elevation of Bim but not BMF protein levels on depletion of HDAC4. ( e ) RelB-p52 regulation of miR-221 in MM cells. RNA from JJN3 cells infected with lentiviruses expressing Control-sh RNA or sh-RNAs targeting RelB, NF-kB2 or HDAC4 were analysed by quantitative PCR for miR-221 expression. Note the down regulation of miR-221 on RelB or NF-κB2 depletion but not on HDAC4-depletion. ( f ) Exogenous miR-221 prevents elevation of BMF protein levels in RelB-depleted cells. JJN3 cells infected with control or miR-221 expressing lentiviruses were superinfected with lentiviruses expressing control-Sh RNA or sh-RNA targeting RelB. Whole cell lysates were analysed by immunoblotting for the indicated proteins. Note the elevation of Bim protein levels in RelB depleted cells in both control and miR-221 overexpressing cells, whereas BMF protein levels were increased only in RelB depleted control but not in miR-221 over expressing cells. *non-specific band. Error bars indicate s.d. n =3. Representative figures from 3 experimental replicates are shown. Full size image Regulation of an oncomir miR-221 by RelB-p52 in MM In line with its recruitment to BMF and Bim gene promoters, depletion of HDAC4 or treatment with the HDAC inhibitor TSA resulted in elevated mRNA levels of both BMF and Bim ( Fig. 4c , Supplementary Fig. 4b,c ). Surprisingly, depletion of HDAC4 resulted in the elevation of Bim ( Fig. 4d , Supplementary Fig. 4d ) but not BMF protein levels ( Fig. 4d ) although mRNA levels of both genes were elevated. Two different sh-RNAs targeting HDAC4 were employed and obtained similar results ( Fig. 4d ). It was previously shown that miR-221 targets BMF mRNA and impairs its translation [41] . Moreover, miR-221 levels were elevated in MM cells [42] and suppression of miR-221 resulted in significant anti-tumour activity in MM [43] . Therefore, we tested whether miR-221 levels are regulated by RelB-p52 but not HDAC4 in MM. To this end, we analysed the levels of miR-221 in control, RelB-, p52- and HDAC4-depleted MM cells by quantitative PCR and found that depletion of RelB or p52 results in reduced miR-221 expression whereas HDAC4 depletion had no affect ( Fig. 4e ). We then tested whether RelB regulate the miR-221 by directly binding to its promoter region. By employing ChIP assay we found that RelB is recruited to a region (−1,222 to −911) within the miR-221 promoter ( Supplementary Fig. 4e ). Further, we cloned a 2.5-kb promoter region of miR-221gene into pGL2-basic luciferase vector and found that cotransfection of both RelB and p52 results in significant induction of the miR-221 promoter activity ( Supplementary Fig. 4f ). To confirm that miR-221 affects BMF protein levels in MM, we infected MM cells either with control virus or a lentivirus expressing miR-221 and found that overexpression of miR-221 results in reduced BMF levels ( Supplementary Fig. 4g ). We then investigated whether reduction in miR-221 levels accounts for the increased BMF protein levels in RelB-depleted cells. To this end, we depleted RelB in control or miR-221 overexpressing MM cells and found that exogenous miR-221 prevented increase in BMF but not Bim protein levels upon RelB-depletion ( Fig. 4f ). Collectively, these results indicate that RelB-p52 contributes to a two-step regulatory mechanism for BMF repression that involves transcriptional and translational regulation (see model in Fig. 8 ). HDAC4 is essential for MM survival and growth To confirm that HDAC4-regulation of Bim and BMF genes is physiologically relevant for MM cell survival we analysed the apoptotic response to HDAC4-depletion in several genetically diverse MMCLs. As indicated in Fig. 5a and Supplementary Fig. 5a , depletion of HDAC4 resulted in apoptosis of various MMCLs. Importantly, HDAC4-depletion completely impaired xenograft growth of human myeloma tumours in vivo in nude mice ( Fig. 5b ). Moreover, HDAC4-depletion also impaired colony-forming ability of MM progenitor cells in semisolid methyl-cellulose cultures ( Fig. 5c , Supplementary Fig. 5b ). These results indicate that similar to RelB–p52, HDAC4 is essential for the survival of several genetically diverse MM cells and for MM tumour growth in vivo . 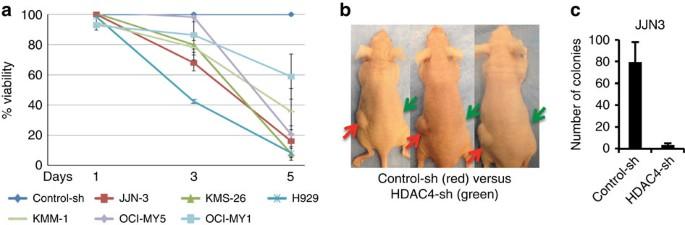Figure 5: HDAC4 is essential for MM survival and growth. (a) Several genetically diverse MM cell lines were infected with lentiviruses expressing control-Sh RNA or sh-RNA targeting HDAC4 were analysed for apoptosis by flow-cytometry as explained inFig. 1. (b) HDAC4 is essential for MM tumour growth. JJN3 cells were infected with lentiviruses expressing control-Sh RNA or sh-RNA targeting HDAC4. 2 days later cell viability was measured to be equal among control and HDAC4-depleted cells and 3 × 106cells were subcutaneously injected into nude mice as indicated (Red arrow=Control-Sh and Green arrow=HDAC4-Sh). Tumour growth was followed for about 3 weeks. Note the complete lack of tumour growth in the absence of HDAC4. Representative figure from 3 experimental replicates (n=3 in each experiment) is shown. (c) HDAC4 is essential for MM tumour progenitor cell growth. JJN3 cells were infected with lentiviruses expressing control-Sh RNA or sh-RNA targeting HDAC4. 24 h later, cells were washed and equal numbers (2000) of cells were seeded into semi-solid methyl-cellulose cultures and the colony formation by MM progenitor cells was followed for about 10 days. Colony numbers were counted on day 10 and plotted as indicated. Error bars indicate s.d.n=3. Representative figures from three experimental replicates are shown. Figure 5: HDAC4 is essential for MM survival and growth. ( a ) Several genetically diverse MM cell lines were infected with lentiviruses expressing control-Sh RNA or sh-RNA targeting HDAC4 were analysed for apoptosis by flow-cytometry as explained in Fig. 1 . ( b ) HDAC4 is essential for MM tumour growth. JJN3 cells were infected with lentiviruses expressing control-Sh RNA or sh-RNA targeting HDAC4. 2 days later cell viability was measured to be equal among control and HDAC4-depleted cells and 3 × 10 6 cells were subcutaneously injected into nude mice as indicated (Red arrow=Control-Sh and Green arrow=HDAC4-Sh). Tumour growth was followed for about 3 weeks. Note the complete lack of tumour growth in the absence of HDAC4. Representative figure from 3 experimental replicates ( n =3 in each experiment) is shown. ( c ) HDAC4 is essential for MM tumour progenitor cell growth. JJN3 cells were infected with lentiviruses expressing control-Sh RNA or sh-RNA targeting HDAC4. 24 h later, cells were washed and equal numbers (2000) of cells were seeded into semi-solid methyl-cellulose cultures and the colony formation by MM progenitor cells was followed for about 10 days. Colony numbers were counted on day 10 and plotted as indicated. Error bars indicate s.d. n =3. Representative figures from three experimental replicates are shown. Full size image Disruption of RelB–HDAC4 complex is toxic to MM cells We next examined whether disruption of the RelB–HDAC4 complex, without knocking down RelB or HDAC4 is sufficient to impair transcriptional repression of Bim and BMF . To this end, we first mapped a 100aa region (aa 125–224) within the N terminus of HDAC4 that is sufficient to bind to RelB and upon overexpression, the Flag-tagged-100aa HDAC4-mimetic polypeptide completely sequestered the endogenous RelB from binding to endogenous HDAC4 in MM cells ( Fig. 6a ). Similarly, upon co-transfection in HEK-293T cells, Flag-tagged 100aa HDAC4-mimetic polypeptide (100aa-H4-Flag) prevented interaction between RelB and full-length HDAC4 ( Supplementary Fig. 6a ). However, 100aa-H4-Flag did not affect interaction of HDAC4 with its known binding partner 14-3-3β ( Supplementary Fig. 6b ) suggesting that the 100aa-H4-mimetic polypeptide specifically disrupts the RelB–HDAC4 complex. We then investigated the impact of RelB–HDAC4 complex disruption on expression of Bim and BMF and found that lentivirus-mediated overexpression of 100aa-H4-Flag resulted in increased mRNA levels of both Bim and BMF in MM cells ( Fig. 6b ). As expected, while the protein levels of Bim were elevated in the presence of 100aa-H4-Flag, BMF protein levels were unaltered ( Fig. 6c ) because HDAC4 is not involved in the regulation of miR-221, which represses BMF mRNA translation as described above. As a control, lentivirus-mediated expression of a Flag-tagged 100aa-GFP-peptide (100aa–GFP–Flag) had no effect on Bim expression ( Supplementary Fig. 6c ). 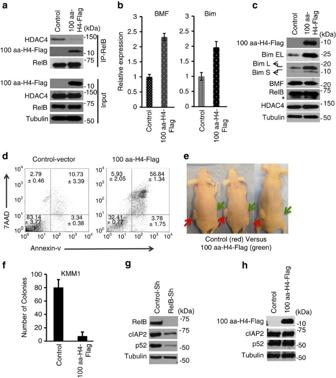Figure 6: Disruption of RelB–HDAC4 complex is toxic to MM cells (a) KMM1 cells were infected with lentiviruses FUGW-Empty or FUGW expressing a Flag-tagged 100aa-HDAC4-mimetic-polypeptide (100aa-H4-Flag) (aa125–224). Twenty four hours later cells were washed, endogenous RelB was immunoprecipitated and RelB–HDAC4 interaction was analysed by immunoblotting as indicated. Note that the 100aa-H4-polypeptide sequesters RelB and completely prevents RelB–HDAC4 interaction. (b) Disruption of RelB–HDAC4 complex results in loss of Bim and BMF gene repression. Total RNA from KMM1 cells infected with control (FUGW-Empty) or FUGW virus expressing the 100aa-H4-Flag was analysed for Bim and BMF levels by quantitative real-time PCR analysis and the relative expression was shown as indicated. (c) Whole-cell lysates from KMM1 cells infected with the indicated viruses were analysed for the indicated proteins by immunoblotting. Note the significant elevation of Bim but not BMF protein levels in the presence of 100aa-H4-Flag polypeptide. (d) KMM1 cells were infected with the indicated viruses and apoptosis was measured 5 days later by flow-cytometry as explained above. (e) JJN3 cells were infected with control (FUGW-empty) or FUGW-100aa-H4-Flag viruses and a day later cells were washed and 3 × 106live cells were subcutaneously injected in to nude mice as indicated. Tumour growth was followed for about 3 weeks. Note the complete block of MM tumour growth in the presence of the 100aa-H4-polypeptide (Green arrows). Representative figure from three experimental replicates (n=3 in each experiment) is shown. (f) KMM1 cells were infected with the indicated viruses and equal numbers (2,000) of cells were seeded into semisolid methyl-cellulose cultures as explained above. Colony numbers were counted after 10 days and plotted as indicated. (g,h) 100aa-H4-Flag impairs transcriptional repression but not transcriptional activation by RelB. RelB-depleted and 100aa-H4-Flag expressing JJN3 cells were analysed for cIAP2 and p52 levels by immunoblotting as indicated. Note the reduced levels of cIAP2 and p52 in RelB-depleted (g) but not in 100aa-H4-Flag expressing cells (h). Error bars indicate s.d.n=3. Representative figures from 3 experimental replicates are shown. Figure 6: Disruption of RelB–HDAC4 complex is toxic to MM cells ( a ) KMM1 cells were infected with lentiviruses FUGW-Empty or FUGW expressing a Flag-tagged 100aa-HDAC4-mimetic-polypeptide (100aa-H4-Flag) (aa125–224). Twenty four hours later cells were washed, endogenous RelB was immunoprecipitated and RelB–HDAC4 interaction was analysed by immunoblotting as indicated. Note that the 100aa-H4-polypeptide sequesters RelB and completely prevents RelB–HDAC4 interaction. ( b ) Disruption of RelB–HDAC4 complex results in loss of Bim and BMF gene repression. Total RNA from KMM1 cells infected with control (FUGW-Empty) or FUGW virus expressing the 100aa-H4-Flag was analysed for Bim and BMF levels by quantitative real-time PCR analysis and the relative expression was shown as indicated. ( c ) Whole-cell lysates from KMM1 cells infected with the indicated viruses were analysed for the indicated proteins by immunoblotting. Note the significant elevation of Bim but not BMF protein levels in the presence of 100aa-H4-Flag polypeptide. ( d ) KMM1 cells were infected with the indicated viruses and apoptosis was measured 5 days later by flow-cytometry as explained above. ( e ) JJN3 cells were infected with control (FUGW-empty) or FUGW-100aa-H4-Flag viruses and a day later cells were washed and 3 × 10 6 live cells were subcutaneously injected in to nude mice as indicated. Tumour growth was followed for about 3 weeks. Note the complete block of MM tumour growth in the presence of the 100aa-H4-polypeptide (Green arrows). Representative figure from three experimental replicates ( n =3 in each experiment) is shown. ( f ) KMM1 cells were infected with the indicated viruses and equal numbers (2,000) of cells were seeded into semisolid methyl-cellulose cultures as explained above. Colony numbers were counted after 10 days and plotted as indicated. ( g , h ) 100aa-H4-Flag impairs transcriptional repression but not transcriptional activation by RelB. RelB-depleted and 100aa-H4-Flag expressing JJN3 cells were analysed for cIAP2 and p52 levels by immunoblotting as indicated. Note the reduced levels of cIAP2 and p52 in RelB-depleted ( g ) but not in 100aa-H4-Flag expressing cells ( h ). Error bars indicate s.d. n =3. Representative figures from 3 experimental replicates are shown. Full size image In line with these results, owing to the elevated levels of Bim, overexpression of the 100aa–H4–Flag, but not a 100aa–GFP–Flag resulted in the apoptosis of MM cells ( Fig. 6d , Supplementary Fig. 6d–h ) and completely prevented xenograft growth of human MM tumours in vivo in nude mice ( Fig. 6e ). Moreover, similar to RelB- or HDAC4-depletion, overexpression of the 100aa-H4-mimetic polypeptide also prevented colony formation by the MM progenitor cells ( Fig. 6f ). Importantly, the 100aa-H4-mimetic polypeptide selectively impaired the transcriptional repressive function of RelB–HDAC4 complex without affecting the transcriptional activation by RelB as indicated by a requirement of RelB for cIAP2 and p52 expression and normal expression of cIAP2 and p52 in 100aa-H4-mimetic polypeptide-expressing cells ( Fig. 6g,h ). Thus, targeting the repressive RelB–HDAC4 complex using the 100aa-H4-mimetic polypeptide is highly toxic to MM cells, an observation that has high translational implications for MM treatment. Constitutive phosphorylation of RelB in MM Since, NIK activity did not correlate with the requirement for RelB-dependent survival in several MMCLs ( Fig. 1a , Supplementary Fig. 1b ), we analysed other potential RelB-activating signals by investigating the phosphorylation status of RelB in MMCLs and primary human MM cells. Using a Serine-573 phospho-RelB-specific antibody we found that in most MMCLs including the NIK low MM cells, RelB is constitutively phosphorylated ( Fig. 7a , Supplementary Fig. 7a ). Moreover, RelB is highly phosphorylated in primary human patient derived MM cells but not in normal B-cells purified from healthy donors ( Fig. 7b ). Interestingly, phospho-RelB was primarily localized to the nucleus in contrast to total RelB, which is distributed in both cytoplasmic and nuclear compartments ( Fig. 7c ). To investigate the physiological relevance of RelB-phosphorylation to MM cell survival, we analysed whether phospho-RelB is essential for repression of Bim. To this end, by employing ChIP analysis, we found that phospho-RelB is readily recruited to the Bim promoter ( Fig. 7d ). We then expressed wild-type (WT) or phospho-mutant RelB (S-573-A) in MM cells and found that moderate expression of exogenous WT-RelB represses Bim whereas expression of phospho-mutant RelB results in elevated levels of Bim indicating that phospho-RelB is essential for Bim repression ( Supplementary Fig. 7b and Fig. 7e,f ). 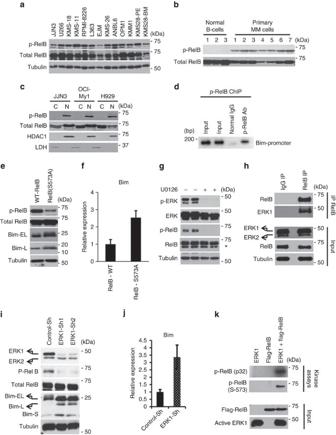Figure 7: ERK1 dependent RelB phosphorylation and Bim repression. (a) Whole cell lysates from the indicated MM cell lines were analysed for phospho (S573) and total RelB by immunoblotting as indicated. (b) Whole-cell lysates from CD138+enriched primary MM cells from human patients and CD19+enriched B-cells from normal healthy human donors were analysed for phospho or total RelB by immunoblotting as indicated. (c) Nuclear (N) and cytoplasmic (C) extracts were analysed for the indicated proteins by immunoblotting. (d) Recruitment of phospho-RelB toBimpromoter was analysed by ChIP analyses as described above inFigure 2, using normal IgG or Phospho RelB specific antibodies and specific primers corresponding toBimpromoter (e,f) Whole-cell lysates (e) and total RNA (f) from JJN3 cells expressing WT-RelB or S573A-RelB (phospho-mutant RelB) were analysed for the indicated proteins by immunoblotting and by quantitative PCR respectively. (g) JJN3 cells were incubated with MEK inhibitor U0126 for 6 h and the whole-cell lysates were analysed for the indicated proteins by immunoblotting. (h) ERK1 interacts with RelB. Endogenous RelB from JJN3 whole cell lysates was immunoprecipitated and probed for the indicated proteins by immunoblotting (i) JJN3 cells were infected with lentiviruses expressing control-Sh RNA or two different sh-RNAs targeting ERK1. Two days later, whole-cell lysates were analysed for the indicated proteins by immunoblotting. Note the complete block of RelB-phosphorylation and elevated levels of Bim in the absence of ERK1. (j) Total RNA from Control-Sh RNA or ERK1-Sh RNA expressing cells was analysed by quantitative PCR for Bim levels. Relative expression of Bim was plotted as indicated. (k) ERK1 is a novel RelB-kinase. Purified Flag-RelB and purified active ERK1 were either co-incubated or incubated separately in a kinase assay in the presence of 32p-ATP (upper lane) or cold ATP (Lower lane). RelB phosphorylation was analysed by the incorporation of 32p (upper lane) or by immunoblotting using anti-phosphoRelB antibody specific to S-573 (lower lane). Inputs were shown in the lower panel. Error bars indicate s.d.n=3. Representative figures from three experimental replicates are shown. Figure 7: ERK1 dependent RelB phosphorylation and Bim repression. ( a ) Whole cell lysates from the indicated MM cell lines were analysed for phospho (S573) and total RelB by immunoblotting as indicated. ( b ) Whole-cell lysates from CD138 + enriched primary MM cells from human patients and CD19 + enriched B-cells from normal healthy human donors were analysed for phospho or total RelB by immunoblotting as indicated. ( c ) Nuclear (N) and cytoplasmic (C) extracts were analysed for the indicated proteins by immunoblotting. ( d ) Recruitment of phospho-RelB to Bim promoter was analysed by ChIP analyses as described above in Figure 2 , using normal IgG or Phospho RelB specific antibodies and specific primers corresponding to Bim promoter ( e , f ) Whole-cell lysates ( e ) and total RNA ( f ) from JJN3 cells expressing WT-RelB or S573A-RelB (phospho-mutant RelB) were analysed for the indicated proteins by immunoblotting and by quantitative PCR respectively. ( g ) JJN3 cells were incubated with MEK inhibitor U0126 for 6 h and the whole-cell lysates were analysed for the indicated proteins by immunoblotting. ( h ) ERK1 interacts with RelB. Endogenous RelB from JJN3 whole cell lysates was immunoprecipitated and probed for the indicated proteins by immunoblotting ( i ) JJN3 cells were infected with lentiviruses expressing control-Sh RNA or two different sh-RNAs targeting ERK1. Two days later, whole-cell lysates were analysed for the indicated proteins by immunoblotting. Note the complete block of RelB-phosphorylation and elevated levels of Bim in the absence of ERK1. ( j ) Total RNA from Control-Sh RNA or ERK1-Sh RNA expressing cells was analysed by quantitative PCR for Bim levels. Relative expression of Bim was plotted as indicated. ( k ) ERK1 is a novel RelB-kinase. Purified Flag-RelB and purified active ERK1 were either co-incubated or incubated separately in a kinase assay in the presence of 32p-ATP (upper lane) or cold ATP (Lower lane). RelB phosphorylation was analysed by the incorporation of 32p (upper lane) or by immunoblotting using anti-phosphoRelB antibody specific to S-573 (lower lane). Inputs were shown in the lower panel. Error bars indicate s.d. n =3. Representative figures from three experimental replicates are shown. 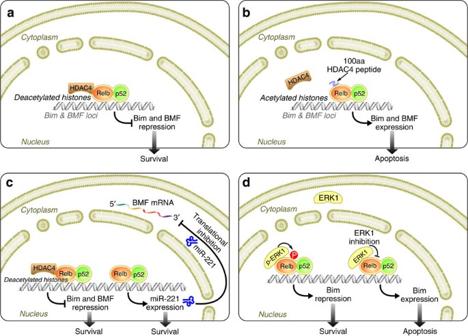Figure 8: A Model that integrates HDAC4, p52, RelB and ERK1 into MM cell survival. (a) A novel HDAC4–RelB–p52 complex is frequently formed in MM cells that maintains deacetylated state of histones aroundBimandBMFloci leading to transcriptional repression of bothBimandBMFgenes and promotes MM cell survival. (b) Disruption of RelB–HDAC4 complex by a HDAC4-mimetic-peptide results in impaired repression ofBimandBMFloci leading to enhanced expression of Bim and BMF and apoptosis of MM cells. (c) RelB-p52 repress BMF in a two-step mechanism: 1) Transcriptional repression ofBMFpromoter by the HDAC4–RelB–p52 complex that maintains deacetylated state of histones and 2) Regulation of miR-221 expression by RelB-p52. RelB-p52 induced expression of miR-221 will further repress the BMF by impairing the translation of BMF mRNA. (d) ERK1 is a novel RelB-kinase. In MM cells RelB and ERK1 constitutively interact with each other. ERK1 is constitutively in an active form that phosphorylates RelB leading to nuclear accumulation of phospho-RelB and phospho-RelB dependent repression ofBimpromoter. ERK1 might phosphorylate RelB in the cytoplasm, nucleus or on the promoter itself. Specific inhibition of ERK1 is sufficient to block RelB-phosphorylation leading to enhanced Bim expression and MM cell apoptosis. Full size image Figure 8: A Model that integrates HDAC4, p52, RelB and ERK1 into MM cell survival. ( a ) A novel HDAC4–RelB–p52 complex is frequently formed in MM cells that maintains deacetylated state of histones around Bim and BMF loci leading to transcriptional repression of both Bim and BMF genes and promotes MM cell survival. ( b ) Disruption of RelB–HDAC4 complex by a HDAC4-mimetic-peptide results in impaired repression of Bim and BMF loci leading to enhanced expression of Bim and BMF and apoptosis of MM cells. ( c ) RelB-p52 repress BMF in a two-step mechanism: 1) Transcriptional repression of BMF promoter by the HDAC4–RelB–p52 complex that maintains deacetylated state of histones and 2) Regulation of miR-221 expression by RelB-p52. RelB-p52 induced expression of miR-221 will further repress the BMF by impairing the translation of BMF mRNA. ( d ) ERK1 is a novel RelB-kinase. In MM cells RelB and ERK1 constitutively interact with each other. ERK1 is constitutively in an active form that phosphorylates RelB leading to nuclear accumulation of phospho-RelB and phospho-RelB dependent repression of Bim promoter. ERK1 might phosphorylate RelB in the cytoplasm, nucleus or on the promoter itself. Specific inhibition of ERK1 is sufficient to block RelB-phosphorylation leading to enhanced Bim expression and MM cell apoptosis. Full size image ERK1 is a novel RelB kinase The physiological importance of RelB-phosphorylation has not been well studied especially in the context of tumour growth and the only known kinase for RelB at Ser-573 to date is GSK3β (ref. 44 ). It has been previously shown that GSK3β-dependent RelB-phosphorylation results in the degradation of the latter [44] . However, we found that RelB is phosphorylated in a GSK3β-independent manner ( Supplementary Fig. 7c ) and that phospho-RelB-S573 is quite stable and has a nuclear function in the regulation of Bim gene in MM cells. Therefore, we sought to identify a novel RelB-kinase in MM by pharmacologically inhibiting several potential kinases and found that inhibition of the MAP kinase MEK-ERK pathway completely abolished RelB-phosphorylation in several MM cells including the NIK low cells ( Fig. 7g , Supplementary Fig. 7d,e ). MEK–ERK inhibition however, did not affect p100 processing ( Supplementary Fig. 7d ). Motif-Scan analysis suggested that ERK1 could be a potential RelB-kinase. Therefore, we investigated whether endogenous ERK1 and RelB interact with each other and found that RelB constitutively interacts with ERK1 in MM cells ( Fig. 7h ). Further, sh-RNA-mediated depletion of ERK1 resulted in complete abolishment of RelB-phosphorylation leading to elevated levels of Bim ( Fig. 7i,j ). To ensure that ERK1 directly phosphorylates RelB, we incubated purified active ERK1 with purified Flag-tagged RelB in a kinase assay and found that ERK1 directly phosphorylates RelB ( Fig. 7k ) suggesting that RelB is a direct substrate for the kinase ERK1. Active ERK is known to regulate transcription factors in the nucleus [45] and we detected significant amounts of nuclear phospho-ERK1 in MM cells ( Supplementary Fig. 7f ). Finally, in line with its requirement to phosphorylate RelB and repress Bim , depletion of ERK1 resulted in significant apoptosis of MM cells ( Supplementary Fig. 7g ). These results indicate that ERK1 is a RelB-kinase and that ERK1-dependent RelB phosphorylation is a novel RelB regulatory mechanism that plays a critical role in Bim repression and MM cell survival. While previous work from Neil Perkins group has elegantly demonstrated transcriptional repression by NF-κB [46] , [47] , whether NF-κB maintains protumorigenic repressive chromatin has not been established. We showed here an important role for transcriptional repression by RelB-p52 in the operation of novel survival strategies in MM. Further, we identified that RelB–p52, by forming a transcriptional repressive complex with HDAC4, maintains repressive chromatin on BMF and Bim gene promoters. RelB-p52, however, did not significantly influence the expression of most anti-apoptotic genes belonging to the Bcl2 family. In line with this, co-depletion of Bim and BMF was sufficient to rescue RelB-depleted MM-cells from apoptosis indicating that Bim and BMF repression is central to the survival and growth of MM. Our data indicated that formation of HDAC4-RelB complex is essential for MM cell survival and that disrupting this complex by the 100aa-H4-polypeptide without knocking down individual molecules was sufficient to derepress Bim and BMF genes, prevent MM tumour growth, and impair colony formation by MM-progenitor cells. ( Fig. 6 , see also model in Fig. 8 ). Thus, the 100aa-H4-mimetic polypeptide has got high translational significance in MM. Although blocking the NF-κB pathway has been previously shown to prevent tumour growth [23] , [48] , complete block of classical or alternative pathways by IKKβ-inhibitors [49] or NIK inhibitors [50] , respectively, will have toxic side effects as both these pathways have important functions in normal homeostasis [8] . Therefore, targeting a downstream NF-κB complex that is important for tumour growth such as the HDAC4–RelB complex might be beneficial. However, complete knockdown of RelB or HDAC4 will likely induce toxic side effects as both these molecules are important for normal homeostasis [8] , [51] . Therefore, development of an approach to selectively target distinct molecular complexes without affecting other complexes formed by the same molecules would be of significant therapeutic advantage. The 100aa-H4-polypeptide described here, selectively targeted the transcriptional repressive complex formed by RelB (RelB–HDAC4) without affecting the transcriptional activation by RelB ( Fig. 6 ) and did not interfere with the interaction of HDAC4 with other partners such as 14-3-3β ( Supplementary Fig. 6b ). Thus, the 100aaH4-polypeptide while being highly toxic to MM cells, is expected to have limited side effects due to its specificity towards HDAC4–RelB complex. We propose that this peptide can be further developed into a novel therapeutic approach for MM and can be used either alone or in combination with other potent anti-MM drugs such as Bortezomib. While activation of RelB–p52 was known to be regulated by NIK, we showed here that some basal levels of nuclear RelB–p52 were sufficient for the survival of most MMCLs including H929 and KMS-28BM in which NIK levels were invisible ( Supplementary Fig. 1b ). Although NIK stabilization is required for receptor-induced processing of p100 and activation of RelB–p52 (refs 25 , 26 ), some basal processing of p100 and nuclear translocation of RelB–p52 does occur under resting conditions in the absence of visible NIK levels as well as in the absence of functional NIK [25] , [28] . Moreover, basal cytoplasmic–nuclear shuttling of NF-κB family members has been reported to contribute to the basal transcriptional regulation of target genes by NF-κB [52] . In line with this, our data clearly indicated that RelB binds to Bim promoter not only in NIK high MMCLs with stabilized NIK (JJN3) but also in NIK low MMCLs without visible NIK levels (KMS28-BM and H929 and so on; Fig. 2 ; Supplementary Figs 1b and 2j ) suggesting that transcriptional repression by basal levels of nuclear RelB-p52 plays an important role in MM cell survival. Nevertheless, in addition to Bim and BMF repression by basal RelB-p52, it is likely that NIK-dependent RelB-p52 activation may have other protumorigenic functions in MM that need to be further investigated. Current therapeutic approaches for MM are not very effective due to development of resistance to drugs such as Bortezomib [34] , [35] . While the mechanism of resistance development to Bortezomib is not clear, it was suggested that MM progenitor cells that are CD138 − and XBP1s − are relatively resistant to Bortezomib [39] , [40] . It is well established that to completely eradicate tumour growth, elimination of tumour progenitor cells is necessary [53] , [54] . The common requirement of RelB–p52 for the survival of genetically diverse MMCLs, Bortezomib-resistant cells as well as MM progenitor cells, suggest that RelB-p52 are excellent molecular targets to develop more affective therapeutic approaches for MM. In contrast to other NF-κB family members, little is known about post-translational modifications of RelB. Importantly, the physiological significance of RelB-phosphorylation has been elusive especially because a previous study based on analysis of T-cells reported that similar to the IκB molecules, the consequence of RelB-S573 phosphorylation is its degradation suggesting an inhibitory role for RelB [44] , [55] . On the contrary our results presented here indicate that phospho-RelB-S573 in MM cells is not degraded and is required for Bim -repression ( Fig. 7 ), suggesting that S573-RelB-phosphorylation is essential for MM cell survival. Further, we reported here that RelB-S573 phosphorylation is ERK1 dependent but GSK3β independent in MM cells ( Fig. 7 , Supplementary Fig. 7 ). Identification of ERK1 as a RelB kinase in this study, is of high physiological significance because MEK-ERK pathway is activated in several tumours and inflammatory disorders and it remains to be studied whether ERK1–RelB cross-talk plays a critical role in those disorders as well, particularly with the tumours associated with oncogenic Ras mutations. Moreover, both the MAPK–ERK pathway and NF-κB pathways are simultaneously activated by several signalling pathways during inflammatory/immune responses. Thus, it is of significant interest to further study the physiological impact of ERK1–RelB cross-talk on normal homeostasis of the immune system as well as other disorders associated with these pathways. While NF-κB activation is predominantly regulated by IKK or NIK-dependent nuclear translocation and DNA-binding, once in the nucleus, it is not clear how different genes are distinctly regulated by different NF-κB complexes. The ERK1-RelB cross-talk presented here may contribute to specific regulation of distinct target genes by RelB and may also determine the protumorigenic RelB-dependent gene regulatory signature. Collectively, the ERK1-dependent RelB-S573-phosphorylation and Bim repression reveals a novel RelB-regulatory mechanism that may offer an explanation for the NIK-independent requirement of RelB for MM cell survival. Panobinostat (LBH-589), a pan-HDAC inhibitor has been used in combination with Bortezomib in MM therapy [56] , [57] and has recently been approved by the FDA for its clinical use against MM. However, it is not clear which HDAC is commonly required for survival of genetically diverse groups of MMCLs. Panobinostat, in addition to other HDACs, also targets HDAC4 and restricts it to the cytoplasm [58] . Our data presented here identified HDAC4 as a critical mediator of MM cell survival by forming the transcriptional repressive complex HDAC4–RelB–p52 that has a nuclear function in the repression of Bim and BMF genes. Importantly, similar to RelB–p52, depletion of HDAC4 or disruption of the HDAC4–RelB complex by the 100aa-H4-mimetic polypeptide has impaired colony formation by MM tumour progenitor cells and blocked MM tumour growth in vivo . Thus, selective targeting of HDAC4 instead of using pan-HDAC inhibitors might provide a more specific and less toxic therapy for MM. Collectively, the work presented here establishes the physiological significance of transcriptional repression by RelB-p52 in MM tumour survival and growth, and identifies potential translational approaches for targeting this mechanism such as disruption of the HDAC4–RelB complex and inhibition of RelB phosphorylation by employing MEK–ERK1 inhibitors. We propose that targeting of HDAC4–RelB–p52 alone or in combination with Bortezomib treatment and/or MEK-ERK inhibitors might offer a highly specific and effective therapeutic approach for the treatment of most MM subgroups. Altogether, this study significantly advances our understanding of regulation of alternative NF-κB (RelB–p52) by a previously unknown cross-talk with the MAPK–ERK pathway and advances our efforts to develop novel therapeutic strategies for MM treatment. Cell culture and cell lines MMCLs [23] , [24] , [59] , [60] used in this study were obtained from Dr Walter M Kuehl (NIH) and from Dr Leif Bergsagel (Mayo Clinic) labs. NHL cell lines [50] used in this study were obtained from Dr Brian A Lewis Lab (NIH). Cells were cultured in RPMI-1640 medium containing L-glutamine (Cellgro) supplemented with 10% fetal bovine serum (FBS; Sigma) and 1% Pen Strep (Gibco). HEK-293T cells were cultured in DMEM high glucose medium (Cellgro) supplemented with 10% FBS (Sigma), 1% Pen Strep (Gibco) and 1% L -Glutamine (Gibco). Bortezomib-resistant RPMI-8226 cells were generated and maintained as described [61] . On the basis of FISH and reverse transcription (RT)–PCR analysis, MacLeod et al . [62] have reported the H929 cell line on the International Cell Line Authentication Committee (ICLAC) list due to a suspected cross-contamination with K562 cell line in a study by Brietkopf et al . [63] However, Brietkopf et al ., in a subsequent and more detailed study [64] , have shown that their lot of H929 cell line was clearly of plasma cell origin and lacked most of the standard markers for the K562 cell line. Nevertheless, we obtained our MMCLs including the H929 from Dr Kuehl (NIH) and Dr Bergsagel (Mayo Clinic) and hence our study is not affected by the MacLeod’s report. Another cell line RPMI8226 was also reported on the ICLAC list but in this case another cell line COLO-677 was reported to be contaminated by RPMI8226 but not the other way around. Hence our study is not affected by the ICLAC list. Lentiviral transduction and gene silencing pLKO.1 vectors expressing sh-RNAs targeting RelB, NF-kB2, Bim and BMF were obtained from open biosystems. pLKO.1 vectors expressing sh-RNAs targeting HDAC4 and ERK1 were obtained from the Lenti-ShRNA library core facility, Cincinnati Childrens Hospital Medical Center (CCHMC), Cincinnati. The CCHMC lenti-ShRNA core facility has obtained the shRNA libraries from the RNAi Consortium (TRC), which developed genome-wide mouse and human libraries. Specific TRCN clone numbers for sh-RNAs targeting RelB were TRCN0000014713 and TRCN0000014716. Specific TRCN clone numbers for sh-RNAs targeting NF-kB2 were TRCN0000006514 and TRCN0000006512. TRCN clone numbers for sh-RNAs targeting HDAC4 were TRCN0000004829 and TRCN0000314666 and the clone numbers for sh-RNAs targeting ERK1 were TRCN0000006150 and TRCN0000006152. TRCN clone numbers for Sh-RNAs targeting Bim and BMF were TRCN0000001052 and TRCN0000148463 respectively. All the TRCN clones were developed by the RNAi Consortium (TRC) and the information including the Sh-RNA sequence for all the TRCN clones used in this study is available with the Sigma-aldrich company. pLKO.1 lentiviruses were packaged in HEK-293T cells by cotransfecting the pMD2.G (VSV G) envelope plasmid (Addgene # 12259) and the Gag, Pol expressing psPAX2 packaging plasmid (Addgene # 12260) into HEK-293T cells. Cells were cultured for 48 h after transfection and the lentiviral particles were collected from the supernatants and were used to transduce different MM cell lines as described [25] . Thirty-six hours post infection, gene silencing efficiency was analysed by immunoblotting for the respective proteins. Plasmids and transfection pCDNA–RelB, pCDNA–p52 were kindly gifted by Dr Gioacchino Natoli. pBabe–RelB and pBabe–p52 were obtained from Dr Gourisankar Ghosh’s lab. FUGW-EGFP (addgene) was used to clone RelB and or S573A mutant RelB in to BamHI and EcoRI restriction sites upon releasing EGFP. pCMV–beta-gal was purchased from Addgene and pGL2-basic was purchased from Promega. FUGW-Empty vector was constructed by releasing EGFP from the BamHI and EcoRI sites. FUGW vector expressing the 100aa-HDAC4-Flag polypeptide (aa125 to aa224 of HDAC4) was constructed by cloning the 100aa-HDAC4-Flag sequence into the BamHI and EcoRI sites. Similarly 100aa–GFP–Flag polypeptide (aa1 to aa100 of GFP) was cloned into BamHI and EcoRI sites of FUGW vector. FUGW-BMF vector was constructed by cloning human BMF into BamHI and EcoRI restriction sites. Transfection in HEK-293T cells was performed using lipofectamine 2000 (Invitrogen) according to the manufacturer’s recommendations. pCDNA–RelB–S573A was generated by site directed mutagenesis using the following forward and reverse primers 5′- GGG GGC GGC CTC CTA GCC CCG GGG CCT GAA GCC -3′ and 5′- GGC TTC AGG CCC CGG GGC TAG GAG GCC GCC CCC -3′, respectively. Briefly high-fidelity Phusion DNA polymerase was used to amplify the whole parental plasmid and DpnI digested to remove the template. The PCR product was then transformed into NEB10β competent cells and positive clones were sequenced to confirm the mutation. S573A-RelB and WT-RelB were eventually cloned into FUGW-vector into the BamHI and EcoRI restriction sites. pLKO.1 vector over expressing RelB was constructed by cloning RelB cDNA into the EcoRI site. JJN3 cells that moderately overexpress RelB were selected upon culturing infected cells in puromycin for several days. pLKO.1 vector co-expressing sh-RNA (targeting 3′-UTR of RelB) and exogenous RelB was constructed by cloning an expression cassette including ubiquitin promoter, cDNA encoding human RelB and WPRE (Woodchuck Hepatitis Virus Posttranscriptional Regulatory Element) regulatory element into AscI and BamHI restriction sites that are present downstream to the RelB–Sh RNA sequence within the pLKO.1 clone TRCN0000014713. pLenti-III-miR vector expressing miR-221 was purchased from Applied Biological Materials (Cat # mh40296). pLenti-III-Empty vector (control) was generated by releasing the miR-221 sequence. Cell viability assay Viability of cells was analysed by flow cytometry using FACS-Calibur (BD Biosciences), upon staining with Annexin-V and 7AAD or Propidium Iodide (BD Pharmingen) according to the manufacturer’s recommendations. Xenograft tumour growth and colony formation assays Colony formation by MM tumour progenitor cells was analysed by seeding 2000 MM cells in semisolid Iscove’s MDM medium containing Methylcellulose (R&D systems) as per manufacturer’s recommendations. Colony numbers were counted using a light microscope and colony pictures were taken by a Axiovert S100TV microscope (Zeiss). Xenograft tumour studies for MMCLs [60] were performed in 8 weeks old, male athymic nude mice (The Jackson Laboratory) upon subcutaneously injecting 3 × 10 6 cells. Tumour growth was monitored twice a week and tumour volume was measured as described [65] . A sample size of 10 mice was chosen in each case to perform minimal necessary number of experimental replicates and to achieve meaningful conclusions. Mice Mice used in this study were maintained in strict accordance with the recommendations in the Guide for the Care and Use of Laboratory Animals of the National Institutes of Health. The protocol was approved by the Institutional Animal Care and Use Committee (IACUC), University of Cincinnati (Protocol Number: 10-09-09-01). The protocol was in compliance with ethical regulations of the IACUC. Essentially, the IACUC serves as an animal research ethics committee for the welfare of animals. The IACUC plays an important role in ensuring that the animals under its purview are humanely treated. All efforts were made to minimize pain and suffering by appropriately anaesthetising the animals as recommended by the Laboratory Animal Medical Services (LAMS), University of Cincinnati. Primary human cells The primary MM tumour cells from human patients and normal B-cells from healthy donors used in this study were deidentified and the use of such cells was approved by the Institutional Review Board, University of Cincinnati, as a research NOT involving human subjects on 21 December 2011. Nevertheless, written informed consent was obtained from all patients from whom MM cells were obtained. These samples were collected under ethical permission from Oxford Radcliffe Hospital regional ethics committee (REC Ref: 07/Q1607/10). Primary MM tumour cells were isolated and enriched by MACS cell separation kit upon staining with CD138 magnetic beads (Miltenyi Biotec). Normal human B-cells were isolated from peripheral blood upon staining with CD19 magnetic beads (Miltenyi Biotec). The purity was tested to be >90% in both cases. Immunoblot and quantitative PCR methods For whole cell lysates, cells were lysed in Triton-x100 lysis buffer (Tris-HCL, pH 7.4 50 mM, NaCL 150 mM, Triton × 100 1%, EDTA 5 mM) (Boston Bioproducts) containing Complete Mini Protease inhibitors and Phosphatase inhibitors (Roche). Nuclear and Cytoplasmic extracts were prepared as described [27] . Immunoprecipitations were performed by incubating whole cell lysates with the indicated antibodies overnight at 4 °C. Before incubation with specific antibodies, samples were precleared by incubation with Sepharose-6B beads (Sigma-Aldrich) for 1 h at 4 °C and immunoprecipitated with protein G- or protein A-Sepharose (Amersham) for 1 h at 4 °C, after which the beads were washed extensively and the proteins were eluted. The samples whole cell lysates, nuclear/cytosolic extracts and immunoprecipitates were separated by SDS–PAGE and analysed by immunoblotting with antibodies to NF-κB2 (Millipore, #06–413), RelB (Santa Cruz, Sc-226), HDAC4 (Cell Signaling, #5392), acetyl-Histone H3 (Cell Signaling, #9649), HA (12CA5, Roche), Flag (Sigma, F3165), alpha Tubulin (DM-1A, Biogenex), Bim (Cell Signaling #2933), BMF (Cell Signaling, #5889), cIAP2 (R&D systems, #AF8171), IκBα (Santa Cruz, #Sc-371), phospho- IκBα (Cell Signaling, #2859), anti-LDH (Santa Cruz, Sc-33781), anti-HDAC1 (Cell Siganling #5356), β-catenin (Cell Signaling #8480), ERK1 (Cell Signaling, #9102), phospho-ERK1 (Cell Signaling, #9101), phospho-RelB (Cell Signaling, #5025), normal rabbit IgG (Santa Cruz, Sc-2027), normal mouse IgG (Santa Cruz, Sc#2025), HRP-conjugated anti-Rabbit (Cell Signaling #7074), and HRP-conjugated anti-Mouse (Cell Signaling #7076). All the antibodies were used at 1:1,000 dilution. Secondary antibodies were used at 1:5000 dilution. Immunoblots were developed using ECL western blotting substrate (Pierce) and super signal west femto chemiluminescent substrate (Fisher) Blots were cropped to include at least one marker position. Uncropped blots for the main figures were included in Supplementary Fig. 8 . For Quantitative PCR analysis of gene expression, total RNA was isolated from cells using RNeasy Plus kit (Qiagen). First strand cDNA was prepared by Reverse Transcription using iScript select cDNA synthesis kit (Bio-Rad) and quantitative PCR was performed on realplex eppendorf master cycler. Various primers used were: Bim Forward: 5′- TCAACACAAACCCCAAGTCC -3′, Reverse: 5′- TAACCATTCGTGGGTGGTCT -3′; BMF Forward: 5′- GAGGTACAGATTGCCCGAAA -3′, Reverse: 5′- CCCCGTTCCTGTTCTCTTCT -3′;Bad Forward: 5′- CGAGTGAGCAGGAAGACTCC -3′, Reverse: 5′- ATGATGGCTGCTGCTGGT -3′; BOK Forward: 5′- GGCGATGAGCTGGAGATGA -3′, Reverse: 5′- ACCGCATACAGGGACACCA -3′; Bid Forward: 5′- GTGAGGTCAACAACGGTTCC -3′, Reverse: 5′- TATTCTTCCCAAGCGGGAGT -3′; BAK Forward: 5′- GTAGCCCAGGACACAGAGGA -3′, Reverse: 5′- ATAGCGTCGGTTGATGTCGT -3′; Noxa Forward: 5′- AGCTGGAAGTCGAGTGTGCT -3′, Reverse: 5′- TCCTGAGCAGAAGAGTTTGGA -3′, Survivin Forward: 5′- CCAGATGACGACCCCATAGA -3′, Reverse: 5′- GCACTTTCTTCGCAGTTTCC -3′; Bcl-W Forward: 5′- GGCGCACCTTCTCTGATCT -3′, Reverse: 5′- ATCCACTCCTGCACTTGTCC -3′; BclXL- Forward: 5′- ATGGCAGCAGTAAAGACCA -3′, Reverse: 5′- TCCCGGAAGAGTTCATTCAC -3′; Bcl2- Forward: 5′- GGAGGATTGTGGCCTTCTTT -3′, Reverse: 5′- CATCCCAGCCTCCGTTATC -3′. For specific amplification of endogenous Vs exogenous RelB the following primer pairs were used: Endogenous 3′-UTR specific: Forward: 5′- atg ttc ccc aat cat tac cg -3′ reverse: 5′- ctc gcc aag gct gaa tat gt -3′ and Exogenous RelB cDNA specific: Forward: 5′- ccattgagcggaagattcaa -3′ Reverse: 5′- cgcagctctgatgtgtttgt -3′. Quantitative PCR analysis of miR-221 levels was analysed on purifying miR-RNA using a mirvana kit (Qiagen) and the PCR was performed using miR-221 and control RNU-44 specific primers (obtained from Invitrogen) as per the manufacturer’s instructions. Luciferase assay A 2.5 kB Bim , BMF and miR221 gene promoters were PCR amplified using the following primers: Bim-Forward: 5′- GTAGGTACCTTCCGTACGGCAAGACAAG -3′, Bim-Reverse: 5′- GTAGCTAGCGCTCCTACGCCCAATCACT -3′; BMF-Forward: 5′- AATGGTACCAGGATCACTTGAGCCTGGGAGA -3′ and BMF-Reverse: 5′- AACGCTAGCAAAATACGCCTGCTC -3′; miR-221 forward: 5′- CCCTGCTTCACCTTGTAAATTCCACCC -3′ and miR-221 reverse: 5′- TTTCCAGGTAGCCTGAAACCCAGC -3′ and were cloned into pGL2-Basic luciferase reporter plasmid (promega) between the KpnI and NheI sites. The resulting pGL2-Bim-Basic, pGL2-BMF-Basic and pGL2-miR221-basic vectors were used in the luciferase assays as described [66] . Briefly: HEK-293T cells were cotransfected with the pGL2-Bim-Basic or pGL2-BMF-Basic luciferase reporter constructs in combination with the indicated plasmids. All the cells were cotransfected with pCMV- β-gal plasmid as a transfection efficiency control. Twenty four hours post-transfection, cells were lysed in the passive lysis buffer supplied with the luciferase assay substrate (Promega: Cat.# E4550). Lysates were incubated with luciferin and the luciferase activity was measured according to manufacturer’s recommendations using 20/20 n luminometer (Turner Biosystems). β-gal activity was measured by incubating the lysates with 2-Nitrophenyl β-D-galactopyranoside (Sigma: Cat.#N1127-1G) and the β-gal activity was measured using μQuant microplate reader (BioTeK instruments Inc). After normalizing for the β-gal values, relative light units were plotted as a measure for the luciferase activity. Chromatin immunoprecipitation (ChIP) ChIP was performed by using Active motif Chip-IT Express kit following the manufacturer’s protocol. Briefly, cells were incubated with 1% formaldehyde (final concentration) for 10 min at room temperature, followed by incubation with 1.25 mM glycine for 5 min. Cells were then lysed in a low salt buffer (10 mM HEPES pH 7.9, 10 mM KCL, 0.1 mM EDTA, 0.1MM EGTA, 2.5 mM DTT) in the presence of protease inhibitors for 20 min. Nuclei were prepared as described [27] followed by incubation of nuclei in shearing buffer (Active motif). Chromatin of 300–600 bp was prepared by shearing the nuclei for 20 pulses (each pulse for10 s at 30% amplitude), using a Sonica transmembrator Model 500 (Fisher Scientific). Sheared chromatin was incubated with indicated antibodies over night together with 20 ug of salmon sperm DNA, 20 μg of BSA in Triton-x 100 lysis buffer containing protease inhibitors. The reaction mix was incubated for 3 h with Protein G coupled to magnetic beads (Active motif). Protein G Magnetic beads were then washed once with Triton-x 100 lysis buffer, ChIP buffer-1 (Active motif), High salt buffer (Triton-x 100 lysis buffer with 450 mM NaCl final concentration). The beads were further washed twice with ChIP buffer-2 (active motif). Bound chromatin was then eluted by incubating Protein G Magnetic beads with elution buffer for 25 min (active motif), followed by addition of reverse cross linking buffer (active motif). Eluted chromatin was incubated overnight with reverse cross linking buffer at 65 °C to reverse the cross links, followed by Proteinase K (active motif) treatment for 2 h. Proteinase K stop solution (active motif) was added to finally stop Proteinase K. The eluted chromatin was then used for PCR with the indicated primers and the amplified products were analysed on 2% agarose gels. Primers used to amplify a 154-bp (−300 to −146) region of the Bim promoter were: forward—5′- GGTGAGCGGGAGGCTAGGGTAC -3′ and reverse—5′- CAGGCTCGGACAGGTAAAGG -3′. Primers used to amplify a 160-bp (−164 to −4) region of the BMF promoter were: forward—5′- CTT GCA ATG TTT CCA TGG GAA -3′ and reverse: 5′- TAC GCC TGC TCG GGG CAT CCC GCA -3′. Primers used to amplify a 310-bp (−1222 to −911) region of the miR-221 promoter were: forward—5′- AGC CAC AAT AAA ATG GTA GAT TGG -3′ and reverse—5′- CTT TGG ATC ATG AAT TGA CAT T -3′. Kinase assay Active ERK1 (Biovision Catalog#: 7741-5) was incubated in a kinase assay with Flag-tagged RelB purified from HEK-293T cells by immunoprecipitation using α-Flag antibody and by eluting Flag-RelB using 3X Flag-Peptide (Sigma). Kinase assay was performed according to the manufacturer’s instructions (Biovision) in the presence of 32pATP or cold ATP. RelB-phosphorylation was detected by 32p incorporation into Flag-RelB or by immunoblotting with a S-573 phospho-RelB specific antibody. How to cite this article: Vallabhapurapu, S. D. et al . Transcriptional repression by the HDAC4–RelB–p52 complex regulates multiple myeloma survival and growth. Nat. Commun. 6:8428 doi: 10.1038/ncomms9428 (2015).